Direct measurement and modulation of single-molecule coordinative bonding forces in a transition metal complex Coordination chemistry has been a consistently active branch of chemistry since Werner’s seminal theory of coordination compounds inaugurated in 1893, with the central focus on transition metal complexes. However, control and measurement of metal–ligand interactions at the single-molecule level remain a daunting challenge. Here we demonstrate an interdisciplinary and systematic approach that enables measurement and modulation of the coordinative bonding forces in a transition metal complex. Terpyridine is derived with a thiol linker, facilitating covalent attachment of this ligand on both gold substrate surfaces and gold-coated atomic force microscopy tips. The coordination and bond breaking between terpyridine and osmium are followed in situ by electrochemically controlled atomic force microscopy at the single-molecule level. The redox state of the central metal atom is found to have a significant impact on the metal–ligand interactions. The present approach represents a major advancement in unravelling the nature of metal–ligand interactions and could have broad implications in coordination chemistry. Coordination chemistry has emerged as an overwhelmingly active branch of chemistry since Werner published his seminal theory of coordination compounds in 1893 [1] , [2] . A wealth of studies have since then been focused on transition metal complexes, driven by their importance in fundamental chemistry, biochemistry, protein science and industrial catalysis applications [2] . In a coordination compound, a central metal atom is bonded to a surrounding array of coordinating ligands [2] . Coordinative bonding is a special class of chemical covalent bonds, often with strong dipolar nature and complex electronic interactions between central metal atom and ligands. Understanding the nature of the coordinative bonding has ever posed and still remains a tremendous challenge. Extensive investigations on metal–ligand interactions have therefore not surprisingly constituted one of the central themes in coordination chemistry. Nearly all aspects of coordination chemistry, including metal-binding free energies and enthalpies, and bond association/dissociation kinetics so far disclosed are based on average ensemble level information. In the past two decades, the scanning probe microscopies have, however, increasingly enabled non-traditional and single-molecule approaches to physicochemical properties of many important chemical and biological processes [3] , ranging from electron transfer (ET) [4] , [5] , [6] and molecular recognition [7] , [8] to in vivo biochemical processes in a living cell [9] . In terms of transition metal complexes, scanning tunnelling microscopy (STM), particularly electrochemical STM (ECSTM), as an advanced tool has offered detailed mapping of single-molecule conductivity patterns in chemical or/and electrochemical environments [10] , [11] , [12] , [13] . Atomic force microscopy (AFM) imaging and spectroscopy have the power to uncover chemically hidden information that would not be revealed by traditional chemical approaches, for example, mechanical activation of chemical bonds (bond rupture) as well as the influence of stretching forces on chemical reactions [14] , [15] , [16] , [17] , [18] , [19] , [20] , [21] , [22] , [23] , [24] , [25] , [26] , [27] , [28] . A very recent report shows that molecular conductance and Van der Waals forces can also be measured simultaneously by conducting AFM [29] . In comparison to the extensive use of ECSTM in molecular electronics studies [4] , [5] , [6] , electrochemically controlled AFM (ECAFM) has not been exploited nearly as much. This is owing to technical challenges and the use of AFM in liquid environments so far mostly for biochemistry and molecular biology. ECAFM has, however, offered new perspectives in two recent reports. One study by Gaub and coworkers [30] , [31] has shown the feasibility of direct measurement of electrically induced nitrogen–gold bonding via the interaction of DNA fragments with a gold substrate. Another report has demonstrated that significant structural changes of a metalloenzyme can be detected when the enzyme is electrochemically brought from its resting state to its catalytically active state [26] . In the present work, we address direct measurement of single-molecule coordinative bonding forces in a transition metal complex in different oxidation states by ECAFM. Density functional theory (DFT) simulations are also performed to offer a rationale of the experimental observations. Synthesis and surface self-assembly of terpyridine ligands Terpyridine (terpy) was derived with an alkanethiol linker group. Details of the synthesis, chemical structure and molecular dimensions are provided in the Supplementary Information ( Supplementary Fig. S1 ). Thiol derivation enables this ligand to self-assemble onto gold surfaces [10] ( Fig. 1a ) and gold-coated AFM tips. The self-assembled monolayers (SAMs) of the terpy derivative on a Au(111) surface with or without osmium (Os) coordination were systematically studied by electrochemistry, ECAFM and ECSTM. Upon the coordination of Os ions to the immobilized terpy ( Fig. 1a ), the Faradaic signal arising from interfacial ET between Os and the Au(111) electrode was detected directly by cyclic voltammetry ( Fig. 1b ). The linear relation between the peak current and scan rate is a clear indication that the Os ions are bound to the electrode surface via terpy coordination ( Supplementary Fig. S2 ). Reversible interfacial ET was observed, and the ET rate was estimated as 25 s −1 by the Laviron method ( Supplementary Fig. S3 ) [32] , [33] . The surface population of terpy, estimated from the reductive desorption ( Supplementary Fig. S4 ), was controlled by adjusting the terpy solution concentration and adsorption time. For the present purpose, the effective surface coverage of (9.0±0.8) × 10 −11 mole cm −2 (that is, at the submonolayer level) as estimated by the Faradaic charge was used in most measurements. 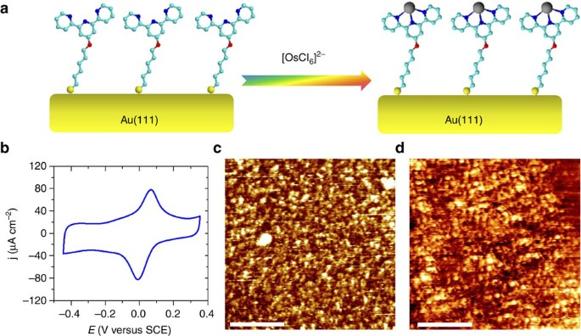Figure 1: Surface self-assembly and characterization of terpy ligands. (a) Schematic illustration of terpy molecules self-assembled on a Au(111) surface and the coordinative binding of Os ions (not drawn to scale). (b) Cyclic voltammogram of Os–terpy SAMs obtained with a scan rate of 1 V s−1. (c) An AFM image and (d) a STM image of Os–terpy SAMs on Au(111) surfaces, recorded by ECAFM and ECSTM in phosphate buffer (10 mM, pH 7.0). The STM image recorded with the key parameters:It=20 pA,Vb=−0.4 V,Ew=−0.02 V (versus SCE). Scan areas: (c) 1,000 nm × 1,000 nm and (d) 100 nm × 100 nm. Scale bar, 250 nm (c) and 25 nm (d). Figure 1: Surface self-assembly and characterization of terpy ligands. ( a ) Schematic illustration of terpy molecules self-assembled on a Au(111) surface and the coordinative binding of Os ions (not drawn to scale). ( b ) Cyclic voltammogram of Os–terpy SAMs obtained with a scan rate of 1 V s −1 . ( c ) An AFM image and ( d ) a STM image of Os–terpy SAMs on Au(111) surfaces, recorded by ECAFM and ECSTM in phosphate buffer (10 mM, pH 7.0). The STM image recorded with the key parameters: I t =20 pA, V b =−0.4 V, E w =−0.02 V (versus SCE). Scan areas: ( c ) 1,000 nm × 1,000 nm and ( d ) 100 nm × 100 nm. Scale bar, 250 nm ( c ) and 25 nm ( d ). Full size image The surface microscopic structures of the terpy-based SAMs were characterized by AFM and STM imaging in electrochemical environment, which were also used in the AFM force spectroscopy. The AFM images ( Fig. 1c and Supplementary Fig. S5 ) show that the apparent height of the Os–terpy complex is about 2 nm, consistent with the molecular dimensions of the half-coordinated complex ( Supplementary Fig. S1 ). In contrast to physical imaging by AFM, in situ STM imaging offers electronic mapping of the molecules and is very sensitive to molecular conductance. Owing to poor conductivity, the terpy SAMs alone show weak STM contrast although the fingerprint features of the SAMs, such as nanoscale pits, are clearly distinguished ( Supplementary Fig. S6 ). The coordination of Os ions to the immobilized terpy results in a dramatic enhancement of molecular conductivity, as shown in Fig. 1d and Supplementary Fig. S7 . STM imaging is thus consistent with the electrochemical observations. While the terpy SAMs are redox inert, the Os–terpy SAMs show reversible and fast interfacial ET. Overall, the electrochemical, AFM and STM characterizations support that the terpy SAMs are formed on Au(111) surfaces and can coordinate to Os. This sets a foundation for single-molecule AFM force spectroscopic analysis. 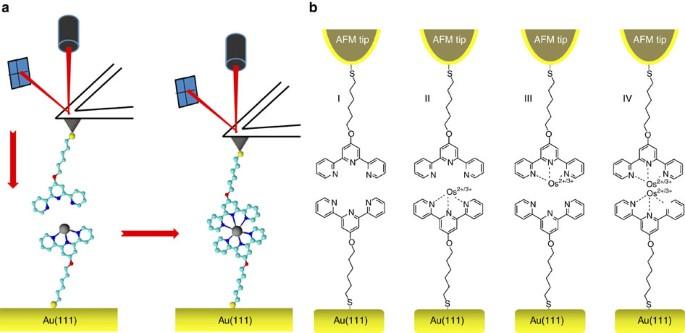Figure 2: AFM force spectroscopy and designed experimental configurations. (a) Schematic illustration of measurement principles of the AFM force spectroscopy for the Os–terpy complex. The cantilever deflection is determined by the position of a reflected laser beam and translated into an interaction force transmitted via the samples. The ligand-functionalized tip approaches the sample and is brought to interact with the sample. (b) Schematic illustrations of four types of experimental configurations for measurements of force spectra: (I) absence of Os ions, (II) Os ions pre-bound to the Au(111) substrate, (III) Os ions pre-loaded on the AFM tip and (IV) Os ions pre-loaded on both the substrate and AFM tip. Direct measurement of single-molecule coordination forces Figure 2a illustrates the working principles of single-molecule AFM force spectroscopy, which is further detailed in Supplementary Fig. S8 . When the AFM tip approaches the sample, tip-bound terpy interacts with Os–terpy on the substrate surface to form the complex ([Os(terpy–(CH 2 ) 6 -S-Au) 2 ] 2+/3+ ). Retraction of the tip results in dissociation of the Os–terpy bond but does not break the Au–S bond, which is much stronger than the coordinative bond as described below. Force–distance curves for the Os–terpy ligand dissociation process can thus be recorded. Figure 2: AFM force spectroscopy and designed experimental configurations. ( a ) Schematic illustration of measurement principles of the AFM force spectroscopy for the Os–terpy complex. The cantilever deflection is determined by the position of a reflected laser beam and translated into an interaction force transmitted via the samples. The ligand-functionalized tip approaches the sample and is brought to interact with the sample. ( b ) Schematic illustrations of four types of experimental configurations for measurements of force spectra: (I) absence of Os ions, (II) Os ions pre-bound to the Au(111) substrate, (III) Os ions pre-loaded on the AFM tip and (IV) Os ions pre-loaded on both the substrate and AFM tip. Full size image To distinguish what AFM force–distance curves actually record, four experimental configurations were designed as illustrated schematically in Fig. 2b . A series of force spectra (several hundreds to thousands force–distance curves) for each configuration were acquired and statistically analysed. 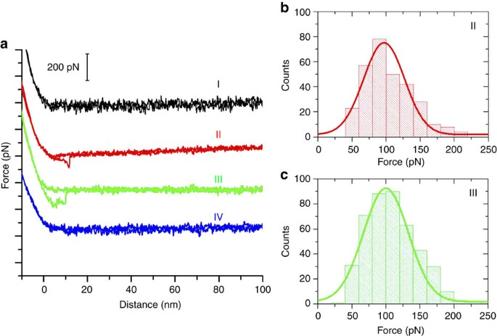Figure 3: Single-molecule force spectra in different experimental configurations. (a) Comparison of typical force-extension curves for the four experimental configurations shown inFig. 2b. The loading rate (LR) of 200 nm s−1was used in recording all the curves. (b,c) The histograms of coordinative force distributions for configurations (II) and (III). The average force is estimated as 97±35 pN (n=300) for configuration II and 100±40 pN (n=432) for configuration III. Figure 3a compares representative force–distance curves at open circuit potentials for the four configurations. In configuration (I), Os ions were absent. When the terpy-C 6 -S-tip was brought in contact with terpy-C 6 -S-Au(111) samples, no specific interaction force was detected ( Fig. 3a(I) ), that is, no force peak feature is observed. Similar observations apply for configuration (IV) ( Fig. 3a(IV) ) where Os ions were pre-loaded on both the AFM tip and Au(111) substrate. In contrast, well-defined force–distance curves were recorded with configurations (II) and (III), and characterized by single force peaks in most cases ( Fig. 3a(II) ). Single force peaks suggest that coordination interaction is most likely detected at the single-molecule level, although they do not exclude several possible interactions occurring simultaneously. The peak widths are in the range of only a few nm reflecting convolution with the cantilever motion ( Fig. 3 ). Multiple peaks are only observed in very few cases, with a probability not more than 5–8% among the featured force spectra. This observation is likely owing to multiple terpy molecules at an AFM tip interacting with the sample occasionally. Owing to low probability and to simplify the data analysis, the force spectra with multiple peaks were not included in our statistical analysis. In addition, it is a challenge to distinguish specific interactions from unspecific ones in some systems. The coordination interaction is regarded as a kind of specific interaction. However, it is unknown to which extent the specificity stands, if compared with the conventional specific interactive systems such as antigen–antibody, substrate–enzyme and ligand–receptor. For example, the same ligand (for example, terpy) can coordinate with various metal ions such as Os, Ru, Zn, Mn and Fe, although with different bonding strength. However, we have designed four experimental configurations as illustrated in Fig. 2b . The results from these configurations show that only configurations II and III yield the featured force spectra, arising from the coordination interactions. There is no (or extremely few) force spectra with features obtained for configurations I and IV from different batches of samples measured. Figure 3: Single-molecule force spectra in different experimental configurations. ( a ) Comparison of typical force-extension curves for the four experimental configurations shown in Fig. 2b . The loading rate (LR) of 200 nm s −1 was used in recording all the curves. ( b , c ) The histograms of coordinative force distributions for configurations (II) and (III). The average force is estimated as 97±35 pN ( n =300) for configuration II and 100±40 pN ( n =432) for configuration III. Full size image Statistical analyses based on hundreds of force curves for each case show that the average force is 100±40 pN ( Fig. 3b ), virtually identical for configurations (II) and (III). This value compares well with that for the terpy–Ru system (95 pN, no potential control) [27] , but is significantly lower than for a covalent bond. For example, previous AFM studies showed that the C–Si bond breaks at 2.0 nN (ref. 17 ), the Si–Si bond at 2.1 nN (ref. 20 ) and the Au–S bond at 2.5 nN (ref. 28 ). The strength of the Os–terpy coordinative bonding is thus about 5% of that for a covalent bond. The coordinative bonds have long been regarded as a special kind of convalent bonds in coordination chemistry. However, it is unknown how strong a coordinative bond should be. The 100 pN force is surprisingly small at first glance. However, the AFM-induced ligand substitution process cannot be regarded solely as a dissociation process. Ligand substitution is instead synchronous dissociation of the outgoing terpy ligand and association of incoming ligands, presumably water molecules to complete the coordination sphere. This notion is supported by the DFT computations, which is described below. Redox-state-dependent coordinative bonding forces ECAFM is capable of controlling the redox state of a transition metal complex and recording force spectra, simultaneously. This ability offers the possibility to explore how the redox state of the metal atom impacts on the bond strength of metal–ligand coordination. In the present case, the Os–terpy SAM is electroactive and its redox state can be controlled by electrochemical potentials applied to the substrate. As recorded by voltammetry (for example, Fig. 1b ), the formal redox potential (that is, in the equilibrium redox state) is around +40 (±5) mV (versus saturated calomel electrode (SCE)). The observed redox potential accords well with that of the redox pair Os 2+/3+ partially coordinated to polypyridine ligands [10] , [11] . A large number of force–distance curves for coordinative bonding at different substrate-working potentials were recorded and statistically analysed. 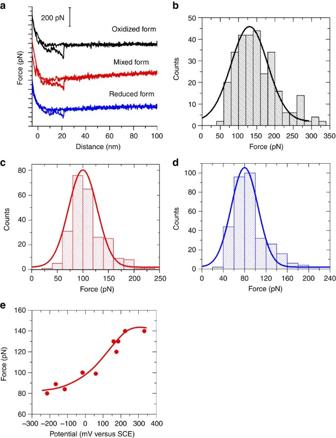Figure 4: Transition metal redox-state-dependent coordinative forces. (a) Comparison of typical force-extension curves for interactions between Os–terpy-C6-S-Au(111) substrates and terpy-C6-S-tips (that is, configuration II) at different working potentials (versus SCE) of +185 mV (fully oxidized state), −15 mV (partially reduced but close to the equilibrium form) and −215 mV (fully reduced form). The LR was 200 nm s−1. (b–d) Corresponding histograms of coordination force distributions. The average force based on statistical analyses is: (b) 130±60 pN (n=292) at +185 mV, (c) 100±30 pN (n=250) at −15 mV and (d) 80±30 pN (n=328) at −215 mV. (e) The dependence of average unbinding forces on the redox states controlled by the working potentials; the data used are the average values of three or four sets of independent experimental measurements. Figure 4a compares typical AFM force spectra recorded at +185, −15 and −215 mV, respectively. The corresponding histograms are shown in Fig. 4b–d . In the fully oxidized form (that is, the working potential applied at +185 mV), the coordinative bonding force was found to be as high as 190 pN, with an average force around 130 pN. The force decreased to about 100 pN, when the Os–terpy complex was partially reduced at −15 mV. The coordinative bonding was further weakened to 80 pN at −215 mV where the complex was in its fully reduced form. More force spectra were recorded at various working potentials and statistically analysed, and the corresponding histograms are shown in Supplementary Fig. S9 . The dependence of the average forces on working potentials is shown in Fig. 4e . The redox-state-dependent transition is thus systematic from the fully reduced form to the fully oxidized form, with a sigmoid-like (that is, ‘ S ’ form) dependence. Figure 4: Transition metal redox-state-dependent coordinative forces. ( a ) Comparison of typical force-extension curves for interactions between Os–terpy-C6-S-Au(111) substrates and terpy-C6-S-tips (that is, configuration II) at different working potentials (versus SCE) of +185 mV (fully oxidized state), −15 mV (partially reduced but close to the equilibrium form) and −215 mV (fully reduced form). The LR was 200 nm s −1 . ( b – d ) Corresponding histograms of coordination force distributions. The average force based on statistical analyses is: ( b ) 130±60 pN ( n =292) at +185 mV, ( c ) 100±30 pN ( n =250) at −15 mV and ( d ) 80±30 pN ( n =328) at −215 mV. ( e ) The dependence of average unbinding forces on the redox states controlled by the working potentials; the data used are the average values of three or four sets of independent experimental measurements. Full size image As the pioneering introduction of the method by Hinterdorfer et al. [34] , the loading rate (LR)-dependent AFM force spectroscopy has offered an effective approach for estimating key parameters that characterize single-molecular interaction events. The method has been used for a wide range of chemical and biological systems [35] , [36] , [37] , [38] , although in some cases the parameters estimated could differ by an order of magnitude even for the same systems. Our AFM measurements were focused on the LR-dependent force spectra at three different oxidation states of the Os–terpy complex. On the basis of statistical analyses of thousands of force spectra, the dependences of the average forces on LRs are presented in Fig. 5 . According to the single barrier model, the correlation between the breaking (or unbinding) force and the LR is rationalized by the approximate form (equation 1) [38] , [39] . 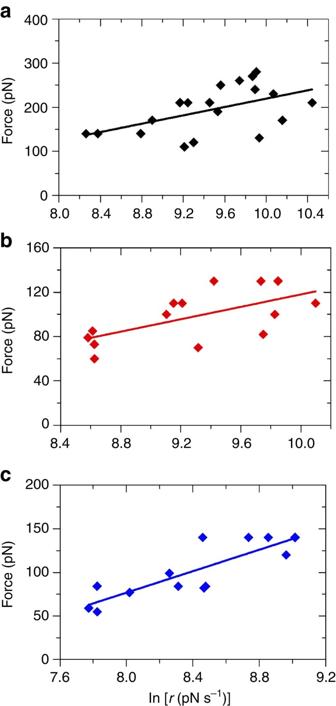Figure 5: Dependence of coordinative unbinding forces on LRs. (a) In the oxidized state (+224 mV versus SCE). (b) In the equilibrium state (+37 mV versus SCE). (c) In the reduced state (−166 mV versus SCE). The solid lines represent the best linear fits to the experimental data. Figure 5: Dependence of coordinative unbinding forces on LRs. ( a ) In the oxidized state (+224 mV versus SCE). ( b ) In the equilibrium state (+37 mV versus SCE). ( c ) In the reduced state (−166 mV versus SCE). The solid lines represent the best linear fits to the experimental data. Full size image where F u is the unbinding force, χ β is the separation distance (energy barrier) from the equilibrium position, r is the LR, k eff is the effective spring constant of the AFM cantilever used, υ is the AFM cantilever retraction velocity, k off is the dissociation kinetic rate constant at zero force, k B is the Boltzmann constant and T is the Kelvin temperature. The parameters χ β and k off can thus be estimated from the slope and intercept of the plot of measured force versus LR, respectively (see for example Fig. 5 ). A recently reported approach was used to estimate the binding kinetic rate constant ( k on ) [37] . The apparent dissociation constant ( K d ) or affinity constant ( K a ) can then be obtained by Equation 2: furthermore, the activation Gibbs energy (ΔE a ) for dissociation of coordination bonding in different redox states is compared, based on their k off values. The smaller the k off value, the higher the dissociation activation free energy. In order to compare the dissociation activation free energy in different redox states, we define the dissociation activation free energy needed for the oxidized form ((ΔE a ) Ox ) as a unit. The relative activation free energy for the equilibrium ((ΔE a ) Eq ) and reduced ((ΔE a ) Re ) states is thus obtained using the following relations [38] . The parameters estimated are summarized in Table 1 . These crucial parameters have re-enforced the systematic effects of the redox state on coordinative interactions observed by direct comparison of forces ( Fig. 4e ), but with more details provided. While all parameters point to the same tendency towards the redox-state effects, their sensitivity and extents could be quite different. The k off values provide a clear distinct by at least a factor of 3 between the fully oxidized and reduced states. The K d (or K a ) values are observably different among the redox states, but they are significantly larger than those obtained by traditional average ensemble approaches to terpy-based transition metal complexes in homogenous solution. There are no K d data available for Os–terpy, but for other transition metals (for example, Mn, Co, Ni, Cd and Fe) K d is in the range of 10 −8 to 10 −3 M, depending on solution pH, ionic strength and the presence or absence of other ligands [40] , [41] . On the one hand, the discrepancy could be in part owing to high uncertainty in the estimates of parameter k on by AFM , as also noted by previous reports on other systems [34] , [35] , [36] , [37] . On the other hand, a direct comparison is not appropriate because the K d values are estimated under very different experimental conditions in AFM and in homogenous solution. In homogenous aqueous solutions, the dissociation of the complex occurs spontaneously in the free state. In the AFM configuration, the Os–terpy complex is immobilized on an Au(111) surface and its dissociation is induced by external mechanic forces (that is, through retraction of the AFM cantilever). Direct comparison for other systems has posed similar challenges [34] , [35] , [36] , [37] , [38] . The relative values of the parameters estimated by AFM force spectroscopy within the same system under different experimental conditions are thus more meaningful. The differences in the dissociation activation free energy are notable but not significant. Nevertheless, in the present case these parameters have offered a possibility of quantitative views on the redox-state-dependent coordinative interactions at the single-molecule level. Table 1 Comparison of the crucial parameters characterizing Os–terpy coordinative interactions in different oxidation states. Full size table The redox-state effects are thus significant. While detailed reasons are not fully understood at present, the different forces reflect higher bonding strengths for Os 3+ than for Os 2+ . Earlier DFT studies for a terpy analogue (2,2′-bipyridine) showed that structural changes caused by the central metal redox state switching are insignificant, when the complex is immobilized on Au(111) surfaces [42] , [43] . The Os–terpy σ bonding might be stronger for Os 3+ than for Os 2+ but this would be counterbalanced in part by relatively poorer π-back donation in the oxidized state. The electronic charge distribution over the complex is different in the two redox states, as charge is relocated from the periphery of the complex to the metal upon oxidation [42] , [43] . Besides, different ligand field stabilization energies (LFSEs) could be a factor. The LFSE is higher for Os 2+ d 6 than for Os 3+ d 5 in fully hexa-coordinated [Os(terpy) 2 ] 2+/3+ . The relatively low oxidation potentials observed suggest, however, that full tri-dentate coordination of both terpy ligands is unlikely. Instead, the coordination of residual H 2 O/OH − ligands could lower the oxidation potential and results in a higher LFSE for Os 3+ than for Os 2+ . To understand the key factors determining the coordinative bonding strength, we performed DFT modelling and computations. DFT computations of coordination pulling force DFT modelling was focused on the different bond rupture forces in the oxidized and reduced forms of the complex and the crucial roles of terpy/H 2 O ligand substitution in the bond rupture process. Before the direct approach to the pulling forces, the potential energy surfaces of the terpy and H 2 O ligand deformation and the electronic structures of the complexes were calculated using the following scheme. The potential energy surface of the terpy ligand was first calculated by rotating two pyridine end units through a whole cycle ( Supplementary Fig. S10 ). The results show that terpy favours a planar geometry, with the two end pyridines in trans- configuration relative to the middle pyridine (that is, N↑N↓N↑). The energy cost for rotating a single pyridine unit, converting the pyridines to the cis configuration (that is, N↓N↓N↓) is about 0.3 eV, consistent with previous reports [44] . Almost the same energy is required to rotate the second pyridine unit. As a consequence, in terms of energy, the cis N↓N↓N↓ configuration is 0.6 e V less stable than the trans- configuration. The conjugation properties are not affected by the orientations of the terpy nitrogen atoms because the energy cost is rooted mainly in steric or electrostatic repulsions between the charged nitrogens. This is supported by Bader analysis ( Supplementary Fig. S11 ). The magnetic properties of the complex were addressed next. Possible low- and high-spin states for Os 2+ (d 6 ) are 0 and 2, and 1/2 and 5/2 for Os 3+ (d 5 ). The energies were calculated for the Perdew–Burke–Ernzerholf (PBE)-relaxed structures of [Os(terpy) 2 (H 2 O) n ] 2+/3+ complexes ( Fig. 6a ) as well as for [Os(terpy)(H 2 O) 3 ] 2+/3+ and [Os(OH 2 ) 6 ] 2+/3+ . Low-spin states were considerably more stable than high-spin states in all cases, with very similar Δ E HS/LS differences for PBE, PBE0 and B3LYP. Δ E HS/LS for [Os(OH 2 ) 6 ] 3+ is calculated as 4.3 to 4.5 eV, which is higher but in the same range as 2.3 eV compared with Os 3+ fully coordinated to two terpy ligands. Bader analysis of Os 2+/3+ (terpy) fragments was used as a reference ( Supplementary Fig. S11 ). The resulting electron distribution is reasonable. For example, all nitrogen donor atoms are negatively charged with a full lone pair, which explains why the trans- configuration is favoured. The charge is acquired mainly from neighbouring carbon atoms. The oxygen donor atoms are also negatively charged, with the bulk of the charge donated by the ligand hydrogen atoms. The positive charge on the hydrogen atoms is fractional, varying from 0.10 to 0.05. Notably the electron distribution at the terpy nitrogen, oxygen and carbon atoms is not significantly perturbed by addition of osmium in either of the two oxidation states. Oxidation of Os 2+ to Os 3+ , however, results in shared electron donation from the metal centre and terpy ligand, that is, with Os further donating half an electron to the ligand. The rest of the holes are distributed in the whole conjugated system, mainly registered as a slight loss of charge on the aromatic hydrogen atoms with the average charge being 0.15 and 0.20 per hydrogen atom, for the Os 2+ and Os 3+ redox states, respectively. 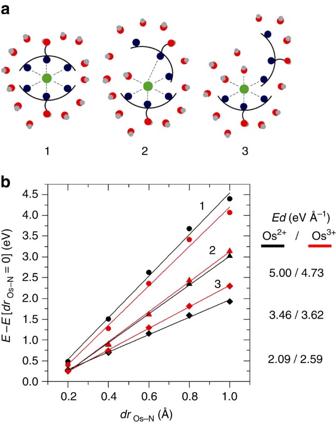Figure 6: DFT simulations of the bond-breaking pulling forces in solution environments. (a) Schematic illustrations of the target bond-breaking systems. Three initial configurations examined in the two oxidation states are: (1) [Os(terpy)2] is osmium in octahedral ligand environment provided by the nitrogen atoms (blue) of two terpy molecules. (2) [Os(terpy)2(H2O)] is coordinated to a second terpy molecule through two nitrogen atoms. The non-bonding group is rotated by about 90°, allowing coordination of a water molecule. (3) [Os(terpy)2(H2O)2] is osmium coordinated to a single nitrogen atom of the second terpy ligand, with two water molecules occupying the coordination sites. The middle pyridine unit of terpy was systematically moved by 0.2 Å increments. At each increment, the Os–N distance (of the middle pyridine unit) was kept fixed and all other degrees of freedom allowed to be relaxed. A notable side reaction was the transfer of a proton from a water ligand to a non-coordinated nitrogen of terpy. (b) Potential energy changes of the simulated bond-breaking systems in aqueous solution. Solid lines are linear best fits to the calculated data for Os2+(black lines) and Os3+(red lines), respectively. The slopes were obtained from these linear fits, and the values are listed in the right panel ofb. It is clear that the Os2+state favours full binding to terpy, but as water occupies coordination sites the terpy–Os3+bond becomes the stronger. It is noted that the energy starts to level off when the Os-to-terpy distance is beyond 1.0 Å. Figure 6: DFT simulations of the bond-breaking pulling forces in solution environments. ( a ) Schematic illustrations of the target bond-breaking systems. Three initial configurations examined in the two oxidation states are: ( 1 ) [Os(terpy) 2 ] is osmium in octahedral ligand environment provided by the nitrogen atoms (blue) of two terpy molecules. ( 2 ) [Os(terpy) 2 (H 2 O)] is coordinated to a second terpy molecule through two nitrogen atoms. The non-bonding group is rotated by about 90°, allowing coordination of a water molecule. ( 3 ) [Os(terpy) 2 (H 2 O) 2 ] is osmium coordinated to a single nitrogen atom of the second terpy ligand, with two water molecules occupying the coordination sites. The middle pyridine unit of terpy was systematically moved by 0.2 Å increments. At each increment, the Os–N distance (of the middle pyridine unit) was kept fixed and all other degrees of freedom allowed to be relaxed. A notable side reaction was the transfer of a proton from a water ligand to a non-coordinated nitrogen of terpy. ( b ) Potential energy changes of the simulated bond-breaking systems in aqueous solution. Solid lines are linear best fits to the calculated data for Os 2+ (black lines) and Os 3+ (red lines), respectively. The slopes were obtained from these linear fits, and the values are listed in the right panel of b . It is clear that the Os 2+ state favours full binding to terpy, but as water occupies coordination sites the terpy–Os 3+ bond becomes the stronger. It is noted that the energy starts to level off when the Os-to-terpy distance is beyond 1.0 Å. Full size image With the electronic and molecular structures available, the Os 2+/3+ pulling energy was simulated in a final stage. Only very small structural differences between the octahedral [Os(terpy) 2 ] 2+ and [Os(terpy) 2 ] 3+ were found. The Os–N bond length at the middle pyridine unit is around 2.01 Å for both redox states. The other two Os–N bond lengths are slightly different, that is, about 2.10 and 2.05 Å for Os 2+ and Os 3+ , respectively. A reference structure was created by relaxing all structures during bond-breaking simulations at a charge of 2.5. The simulations were then started from relaxed geometries of the complexes with varying coordination to terpy and water molecules ( Supplementary Information Fig. S12 ), shifting the middle pyridine unit away within 0.2 Å increments. At each increment, the middle Os–N distance was fixed, while all other degrees of freedom were allowed to relax with the same criteria (0.05 eV Å −1 ). Figure 6a and Supplementary Fig. S13a show three simulated target configurations. The pulling energies ( E − E [dr Os–N =0]) for each configuration were calculated and plotted against the Os–N distance (dr Os–N ) for both redox states. The change in bond length is not shown beyond 1 Å, which is where the terpy–Os bond starts to break. Notably, proton transfer between a water molecule and a terpy nitrogen atom occurs in some cases, giving a step in the potential energy curve. The pulling force was evaluated as the slopes of the best linear fits ( Fig. 6b and Supplementary Fig. S13 ) in the energy profile. The slope is steeper, that is, the pulling force stronger when terpy is fully coordinated to Os 2+ , but this changes dramatically when a single or two water molecules are coordinated ( Supplementary Fig. S13b ). There is then a clear difference in the energy change for the two redox states, with Os 3+ showing considerably stronger bonding and stronger bond force with two water molecules each occupying a coordination site. The calculated forces thus accord qualitatively with the experimental data and is proposed as the most favourable coordination of Os 2+/3+ to terpy under the experimental conditions. It is noted that the quantitative values of the calculated pulling forces are significantly stronger than those observed (that is, nN versus pN). This discrepancy is presumably owing to limitations of the present model. Full coordination would both involve several reorganization steps and more vigorous conditions, and reverse the stability order in favour of Os 2+ . To make the simulations closer to the experimental conditions, a solvation shell of 25–30 water molecules around each complex was added. The water molecules were allowed to relax around the complex ( Supplementary Fig. S12 ) and calculations for both redox states in each configuration were carried out. The relation between the pulling energy and the Os–N distance is shown in Fig. 6b . Compared with vacuum ( Supplementary Fig. S13b ), the addition of a single solvation shell does not change the trend in the relative pulling energy but enhances notably the coordinative bond strength of Os 3+ ( Fig. 6b ). Overall, the DFT simulations suggest the following: the potential surfaces of terpy show that the N↑N↓N↑ configuration is favoured over N↓N↓N↓; the terpy carbon and hydrogen atoms carry a considerable positive charge; beyond 1 Å where the Os–terpy bond breaks, terpy promotes proton transfer from a H 2 O ligand forming a terpy (H + )–OH − ligand pair; the terpy nitrogen atoms are negatively charged, but OH − carries the largest negative charge and interacts more strongly with Os 3+ than with Os 2+ ; and the redox state of Os significantly affects the bonding strength. Os 2+ favours full ligation to terpy, probably owing to larger ligand field stabilization, while Os 3+ favours coordination to one or two terpy ligands, with the other ligand sites occupied by water. Solvation finally enhances the bond strength and pulling force of Os 3+ , and favours ligand binding of Os 3+ over Os 2+ . The latter accords with the experimental data and points to the crucial role of ligand substitution in the pulling process; although as noted, quantitative accordance requires a more comprehensive computational scheme with full incorporation of the solvent. Coordination interaction is a very broad area in chemistry, because more than half of the elements in the periodic table are transition metals, the chemical properties of which are dominated entirely by coordination chemistry. ET and ligand substitution reactions represent the two major classes of reactivity of transition metal complexes with crucial applications in catalysis, molecular electronics and medical chemistry. However, most studies in coordination chemistry, including metal-binding free energies and enthalpies, and bond association/disassociation kinetics, are based on average and ensemble level approaches. While studies on ET of transition metal complexes have been conducted intensively (including single-molecule approaches by STM and related techniques), the present work aims to address the other major class, namely ligand substitution processes at the single-molecule level. Such an approach has not been reported before for ligand–metal interactions in controlled oxidation states of the central metal ion and represents therefore a new exploration in coordination chemistry. In this work, single-molecule force analysis has been achieved by combining several interdisciplinary tools, particularly including ligand design and synthesis, surface self-assembly chemistry, single-crystal electrochemistry, STM imaging, and high-resolution electrochemical AFM force imaging and spectroscopy. The proof-of-concept study is a major focus of this work and has been illustrated well by the Os–terpy systems. The Os–terpy bonds are ruptured at 100±30 pN at open circuit potentials, but at 130±60 pN in the oxidized state of the central metal and at the lower value of 80±30 pN in the reduced state. A remarkable effect of the redox state on the coordinative bonding is thus experimentally observed. Such effects are further detailed by the crucial parameters obtained, relevant to the coordinative bonding and dissociation processes. The different pulling forces in the two oxidation states are rationalized by DFT simulations. The computational procedures are rigorous, though the models used at this stage are relatively crude as the bulk solvation is either disregarded or represented by a single solvation shell only. The emerging pulling forces, however, still disclose clearly the kinematic and electronic nature of the molecular scale pulling events, and the subtle interplay between bond stretching and terpy/H 2 O ligand substitution that controls the process. The latter is a rationale even for the qualitative observations. The quantitative values of the emerging pulling forces are still significantly stronger than those observed (nN rather pN ranges) but the accordance can be expected to change drastically by full scale incorporation of solvent molecular assemblies that incorporate both the dynamics of the accompanying terpy/H 2 O ligand substitution and longer-range solvation. Such a study is in progress. The overall approach demonstrated in this work represents a critical advancement in studying coordination chemistry at the single-molecule level. The observations should add new insight to our understanding of the physicochemical nature of coordinative bonds. The method is expected to apply generally to other transition metal complexes and to impact coordination chemistry and related areas broadly. The AFM force spectroscopy has shown that a metal–ligand coordinative bonding strength is only equivalent to about 5% of that for a covalent bond. This value appears to be surprisingly smaller than expectation from our traditional understanding of metal–ligand interactions in coordination chemistry, where coordinative bonds are considered as a kind of special covalent chemical bonds. These AFM studies have thus raised several interesting but challenging questions such as: how strong a metal–ligand coordination bond should be; what we can learn more about the physicochemical nature of metal–ligand bonding; and how much external conditions such as solution pH, ionic strength and type of transition metals could affect metal–ligand interactions. These questions would promote refined research in the near future, for example, by systematic design and synthesis of various ligands, including mono-, bi-, tri- and multi-binding sites, and by exploring other transition metals as well as introduction of other complementary tools in addition to AFM. Chemicals and reagents Potassium hexachloro-osmate(IV) with high purity (99.99%) from Aldrich and 2,2′: 6′,2′′terpyridine (99%) from Sigma were used as received. Electrolyte solutions (10 mM, pH 7.0) were prepared from KH 2 PO 4 (Sigma-Aldrich, ultrapure 99.99%) and K 2 HPO 4 (Fluka, ultrapure 99.99%). KOH (ultrapure 99.99%) obtained from Sigma-Aldrich was used for the experiments of reductive desorption. Absolute ethanol (EtOH) (Ultrapure, Sigma-Aldrich) was used as a solvent for preparation of terpy solutions. Millipore water (18.2 MΩ) was used throughout. Synthesis and characterization of terpy ligands Terpy with a 4′-(6-acetylthiohexyloxy) linker group ( Supplementary Scheme S1 ), denoted as terpy-C 6 -SAc , was synthesized by reference to a previously reported procedure with modification [45] , [46] , and its structure and chemical properties were systematically characterized. Briefly, to a solution containing compound 1 (1 g, 4 mmol) and anhydrous powdered K 2 CO 3 (1.1 g, 8 mmol) in anhydrous dimethylformamide (20 ml), compound 2 (1.72 g, 7.22 mmol) was added. The solution was heated to 70 °C and stirred for 24 h. The reaction mixture was then cooled down, poured into 100 ml of water and subjected to extraction with dichloromethane three times. The combined organic layers were dried over MgSO 4 , filtered and evaporated under reduced pressure. The spectroscopically clean product was obtained after column chromatography (Al 2 O 3 , Hex:EA (4:1)) and following recrystallization from ethanol (1.3 g, 3.2 mmol, yield: 80%). The chemical reaction is illustrated in Supplementary Fig. S15 . Preparation of terpy monolayers on Au(111) surfaces To prepare the SAMs on substrate Au(111) surfaces and AFM cantilevers, as-synthesized terpy-C 6 -SAc solid was dissolved in ultrapure ethanol (EtOH) to prepare the solutions with the concentration range of 0.05–5 mM. For example, about 5 mg terpy-C 6 -SAc was dissolved in 5 ml EtOH, leading to a concentration of about 0.5 mM. SAMs were formed by immersing the freshly annealed and hydrogen flame-quenched Au(111) substrates and clean gold-coated AFM tips in terpy-C 6 -SAc solutions. After surface modification, the samples were removed from the terpy solution, followed by rinsing with EtOH, Milli-Q water and buffer solution. The samples were then immersed in [OsCl 6 ] 2− containing aqueous solutions (ca. 2 mM) for 3 h. Excess metal compound was removed by rinsing with Milli-Q water. The adsorption time for formation of SAMs on Au(111) surfaces was systematically studied in the range of 2 h to overnight (20 h) with different concentrations of terpy-C 6 -SAc solutions. It was found that the closely packed SAM was formed, only when the terpy-C 6 -SAc concentration is higher than 3 mM with an overnight adsorption. The effective surface concentration of Os–terpy SAMs on Au(111) surfaces is 9.0 (±0.8) × 10 −11 mol cm −2 , which was used in most AFM force spectroscopic measurements. Electrochemistry measurements Cyclic voltammograms were recorded using a 15 ml, three-compartment cell containing phosphate buffer (10 mM, pH 7.0) as electrolyte solution. A freshly prepared reversible hydrogen electrode served as reference electrode and a Pt wire as counter electrode, respectively. The electrolyte solution was degassed with pure Argon for 1 h before electrochemical experiments. All voltammetric measurements were carried out at room temperature (23±2 °C), using an Autolab PGSTAT12 system controlled by the GPES 4.9 software (Eco Chemie, Netherlands). The reference electrode was calibrated against a SCE after each experiment. All electrochemical potentials are reported versus SCE in this work. Experimental procedures for the pretreatment of Au(111) electrodes and single-crystal electrochemical measurements were similar to those used in our previous reports [47] , [48] . STM imaging A PicoSPM (Molecule Imaging, USA) including in situ STM microscope was used. Au(111) disk electrodes (1.2 cm in diameter) were used as in situ STM substrates. A Teflon house-built liquid STM cell, equipped with reference and counter electrodes, was used throughout. The reference electrode was calibrated against a SCE after each experiment. Electrochemically etched Pt/Ir tips (80/20, 0.25 mm in diameter) coated with Apiezon wax served as scanning probe. STM samples were prepared as described above. The detail of experimental procedures on the pretreatment of single-crystal Au(111) substrates and STM imaging can be further referred to our previous reports [47] , [48] . AFM force imaging and spectroscopy AFM imaging and force spectroscopic measurements were carried out using a Scanning Probe Microscope (Model 5500, Agilent Technologies, Chandler, AZ). The Os–Tpy SAMs on Au(111) were imaged in an AAC (Acoustic Alternating Current) mode AFM. Oxide-sharpened Si 3 N 4 probes (Veeco, SNL) with a spring constant of 0.06 N m −1 were applied, mostly suitable for the soft organic adlayers. The typical radius of the SNL tip is about 2–10 nm (Manufacturer’s homepage). Imaging amplitude was set between 2.0 and 2.5 V. The scanner was calibrated using a Veeco 10-μm pitch calibration grating, each square with a 200 nm depth. Scanning speed was 1.6 Hz. For single-molecule force spectroscopy experiments, an in-house-built electrochemical cell was applied for control of the sample potentials. Each individual gold-coated cantilever used was calibrated in solution using the equi-partition theorem before each experiment to obtain the spring constant ( k eff ) (with a typical value around 105 pN nm −1 ). All experiments were carried out at room temperature (23±2 °C) in phosphate buffer (10 mM, pH 7) at a given approaching and pulling speed (for example, 200 nm s −1 ). Totally over 100 gold-coated AFM cantilevers were used in the AFM experiments. The measurements under each experimental condition were repeated at least three times independently with 4–5 tips used in each set of measurements. Different areas of each sample were measured and the areas were changed after about 50 data points were collected for force spectra. DFT modelling and computations All calculations were performed with the real-space Grid-based projector augmented-wave DFT code [49] , [50] . Kohn–Sham states were represented in terms of numerical atom centred orbitals of the double-ζ with polarization quality (DZP). The potential was expressed on a real-space grid with 0.18 (±0.01) Å grid point spacing. The exchange-correlation (xc) energy was approximated using the PBE functional [51] , and the core electrons were described with the PAW method [52] . All structural relaxations were performed with a quasi-Newton scheme at a maximum force tolerance of 0.05 e V Å −1 . Magnetic structures of the two redox states were, furthermore, also analysed with the hybrid-GGA xc-functionals PBE0 [53] and B3LYP [54] . The charge density of the system was calculated using Bader analysis [55] , [56] , which gives localized charges for each atom in the specific system. How to cite this article: Hao, X. et al. Direct measurement and modulation of single-molecule coordinative bonding forces in a transition metal complex. Nat. Commun. 4:2121 doi: 10.1038/ncomms3121 (2013).